The crucial effect of early-stage gelation on the mechanical properties of cement hydrates Gelation and densification of calcium–silicate–hydrate take place during cement hydration. Both processes are crucial for the development of cement strength, and for the long-term evolution of concrete structures. However, the physicochemical environment evolves during cement formation, making it difficult to disentangle what factors are crucial for the mechanical properties. Here we use Monte Carlo and Molecular Dynamics simulations to study a coarse-grained model of cement formation, and investigate the equilibrium and arrested states. We can correlate the various structures with the time evolution of the interactions between the nano-hydrates during the preparation of cement. The novel emerging picture is that the changes of the physicochemical environment, which dictate the evolution of the effective interactions, specifically favour the early gel formation and its continuous densification. Our observations help us understand how cement attains its unique strength and may help in the rational design of the properties of cement and related materials. Cement is the main binding agent of concrete, the most widely used, durable building material. Its production is responsible for 5–8% of anthropogenic carbon dioxide production [1] . In spite of its great practical importance, there is only limited understanding of the fundamental physicochemical processes that give the material its functional properties. At present, this lack of understanding hinders progress towards ‘rational’ cement design, which will be needed for designing novel green formulations with a reduced carbon footprint [2] . For the control of the mechanical properties, calcium–silicate–hydrate (C–S–H), the primary hydration product of Portland cement paste, is of particular importance. C–S–H is known to precipitate as nanoscale particles from the so-called ‘pore solution’ that forms upon mixing the polydisperse cement powder with water. The particles form a highly cohesive gel that acts as a spontaneously densifying glue. The early-stage properties of this gel affect the ultimate strength that cement (and hence concrete) can attain upon hardening at the end of the hydration process [3] , [4] , [5] , [6] . Hence, somewhat surprisingly, the ultimate hardness of cement, which is important for its role in concrete, is determined by the structural properties of the C–S–H gel, that is, of the soft precursor of the final hardened paste. Experiments to probe the gel formation are challenging and therefore few in number [7] , [8] . More work has been carried out, in contrast, on the hardened paste that can be probed by neutron scattering and by atomic force microscopy (AFM) or scanning electron microscopy imaging [9] , [10] , [11] , [12] , [13] . These studies, mainly performed on tri-calcium silicate (the main source of C–S–H in Portland cement and often used as a model system for cement hydration), indicate an amorphous mesoscale organization comprising structural units of locally compact assemblies of calcium–silicate layers with a typical size of ≃ 10 nm (refs 14 , 15 , 16 , 17 ). The main theoretical approaches for modelling the structural evolution of the C–S–H gels have either assumed mesoscale nucleation and growth or nanoscale Diffusion Limited Cluster Aggregation [18] , [19] , [20] , [21] , [22] . Nucleation and growth models are based on the analysis of multicomponent phase diagrams and assume a kinetic evolution scenario to match the one observed in experiments. diffusion-limited cluster aggregation, on the other hand, assumes a completely random, irreversible (and hence purely kinetic) aggregation of colloidal nanoparticles. Calorimetric studies of the (exothermic) C–S–H production show that time evolution of this process is strongly non-monotonic [18] , indicating that the gel growth goes through an acceleration and a deceleration regime, a feature that is difficult to reconcile with the growth kinetics expected for random, fractal aggregation. As a matter of fact, there is at present no theoretical approach that derives, rather than postulates, the scenario that links gel growth to the kinetics and the final morphology and properties of the hardened paste. As a consequence, there is no clear answer to the following basic questions: how can nonequilibrium aggregation, which takes place in a complex and evolving physicochemical environment, still result robustly in reproducible material properties? How does the low-density, fractal structure that is typically produced by irreversible random aggregation evolve to the high density required to give hardened cement its final strength? One key experimental observation is that the effective interactions between the C–S–H units depend strongly on the chemical environment, which evolves in time because of the dissolution of the cement grains and the precipitation of various hydration products [23] . As the chemical composition of the solvent changes, the effective attraction between the nanoscale units increases, mainly because of increasing ionic concentrations in the pore solution. Owing to the presence of multivalent ions, the effective interactions between the nanoscale units show a combination of a short-range attraction and a longer-range electrostatic repulsion, which progressively disappears by the end of the setting [17] , [23] , [24] , [25] , [26] , [27] , [28] . In principle, the dependence of interparticle interactions on the composition of the pore solution could be reproduced using fully atomistic models [29] , [30] . However, simulation of the phase diagram of such models would be prohibitively expensive. Using a coarse-grained ‘implicit solvent’ model that accounts for the time evolution of the interparticle interactions can therefore help investigate how the equilibrium properties and the aggregation of the nanoscale C–S–H clusters evolve in time during hydration. Here we report simulations that allow us to address these open questions and propose a consistent scenario for C–S–H gelation and densification. The computer simulations allow us to identify and characterize both stable and the kinetically arrested states that occur over a range of low to intermediate volume fractions, corresponding to the early stages of cement hydration. Surprisingly, we find that the morphology of the gel, the early development of mechanical strength and the continuous densification of the material are all intimately related to the underlying equilibrium-phase behaviour that is expected for the (evolving) effective interactions between the hydrates. This observation is far from obvious as out-of-equilibrium conditions prevail during gelation and densification. The implication is that the evolution of the material properties strongly depends on the thermodynamic conditions encountered on the path towards hardened cement, and is surprisingly less sensitive than expected to the precise timeline for traversing this path. These findings are important because they indicate that rational design of the properties of cement can be achieved by controlling the effective hydrate interactions along the densification path by a judicious choice of the physicochemical environment and/or the chemical composition of the pore liquid during densification. This would open the way to ‘nanoscale’ engineering of cement, the ultimate ‘bulk’ material. Model and numerical simulations We describe the C–S–H hydrates as colloidal nanoparticles with a diameter σ (ref. 5 ). Without much loss of generality we assume that the interactions between the particles are pairwise additive. The characteristic features of the pair potentials were chosen to agree with experimental observations and atomistic simulations: hydration experiments performed at fixed lime concentrations [31] , nanoindentation experiments in the hardened paste [32] , [33] and atomistic simulations [30] , [34] , [35] are consistent with a model where the hydrate particles of typical size ≃ 10 nm have short-ranged attractive interactions, with a strain at rupture of ≃ 5%. The hydration experiments as well as calculations of ion correlation forces also indicate an intermediate-range residual repulsion (typical screening length for C–S–H in water is ≃ 5 nm); the strength of this repulsion is controlled by the pH, which in turn depends on the lime concentration. The strength of the repulsion decreases in time as the lime concentration increases during the cement hydration. However, the range of the repulsion, which depends on the ionic strength, is roughly constant since the ionic strength is not changing much during lime dissolution [16] , [23] , [36] . We therefore assume a generic model for effective interactions comprising a short-range attractive well and a long-range Yukawa repulsion [37] : r is the interparticle distance and κ is the inverse screening length. The ratio A 1 / A 2 gives the relative strength of attraction and repulsion, while sets the energy scale. Inspired by the experimental observations, we fix two parameter values to γ =12 and κ −1 =0.5 σ and vary A 1 and A 2 in such a manner that the depth of the attraction well in equation (1) is fixed to , whereas the height of the repulsive shoulder, V ( r max ), varies with the ratio A 1 / A 2 . We note that we have used more parameters ( A 1 , A 2 and ) to describe the strength of the potential: two of the three parameters would suffice. However, by defining as the depth of the potential well, it becomes easier to compare results for different potentials with equal strength of attraction. The choice of parameters made in the coarse-grained model allows for a reasonable comparison with the physical systems. With the particle size σ ≃ 10 nm, the position of the minimum and the repulsive shoulder in the interactions are consistent with the experimental results in ref. 31 and recent atomistic simulation studies [35] . The reduced temperature in the simulations is , where T 0 corresponds to the room temperature, that is, to the condition of the AFM experiments, and is the depth of the attractive well and the unit energy in the simulations. Using 2.43 g ml −1 for the density of C–S–H, as in refs 30 , 33 , setting the reduced temperature to T =0.15 roughly corresponds to interparticle forces measured in experiments and simulations. In fact, when considering that the cohesive force measured in the experiments in the early hydration is ≃ 0.5 nN and the contact area between two C–S–H nanoparticles can be estimated ≃ 5 nm 2 , the unit pressure in the simulations corresponds to 20 MPa, which makes the mechanical strength of the gels obtained here comparable to typical values of hydrating cement paste. Moreover, the same coarse-grained model was recently used in simulations of the hardened paste at the end of the hydration [38] . The morphological and mechanical properties obtained in those simulations agree well with the experimental observations, which further supports the choice of the coarse-grained model and interaction parameters in this work. We have studied the phase behaviour of the model hydrate for three typical interaction potentials (shown in Fig. 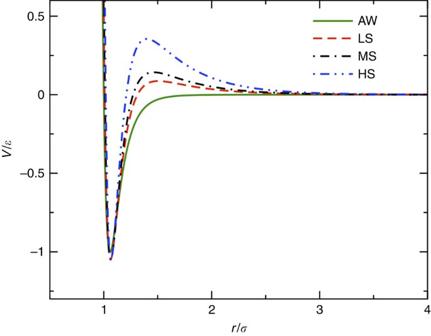Figure 1: Interaction potentials. The curves correspond to LS, MS, HS potentials considered here as a function of the interparticle distancer, plus the purely attractive well case (AW) from ref.58. The corresponding values of the parametersA1andA2, andV(rmax) are listed inTable 1. 1 with the corresponding parameter values listed in Table 1 ) within the regime relevant to the cement hydration (roughly ): ‘high shoulder’ (HS), ‘mid shoulder’ (MS) and ‘low shoulder’ (LS). Figure 1: Interaction potentials. The curves correspond to LS, MS, HS potentials considered here as a function of the interparticle distance r , plus the purely attractive well case (AW) from ref. 58 . The corresponding values of the parameters A 1 and A 2 , and V ( r max ) are listed in Table 1 . Full size image Table 1 Potential parameters. Full size table Numerical simulations of the model allow us to characterize the equilibrium and nonequilibrium states for different densities and values of the reduced temperature 0.1≤ T ≤0.5. The densities are expressed in terms of the particle volume fraction ϕ ≡ πNσ 3 /6 V , where N is the total number of particles and V the volume of the simulation box (see also Methods section). We use these reduced units to facilitate comparison with different real systems that would be characterized by different values of and σ but by roughly similar reduced parameters. Clusters and preferred local packing At low temperatures, that is, for interaction strengths sufficiently larger than k B T , we consistently observe that the particles aggregate into small clusters at low-volume fractions and form a complex gel network upon increasing ϕ , regardless of the differences in the effective potential. However, the shapes and sizes of the clusters, as well as the gel morphology, vary distinctly with the interaction potential (see Fig. 2 ), suggesting that the changes in the effective interactions from HS to LS during the hydration process might drive significant morphological changes in the C–S–H gels. In Fig. 3a we compare the results of the Grand Canonical Monte Carlo (GCMC) and Molecular Dynamics (MD) simulations at low-volume fractions. In GCMC simulations we evaluated the free energy of single clusters of a fixed size (infinitely diluted limit), whereas MD simulations where performed on larger systems ( N =6,912) at finite ϕ and included cluster–cluster interactions. In the case of the HS potential, at low-volume fractions both approaches reveal the existence of small, stable clusters of a well-defined size. At higher ϕ a percolating network forms through growth and aggregation of the clusters. As the height of the repulsive shoulder is decreased (MS), the GCMC data show that the cluster-size distribution at infinite dilution is broader and shifted towards larger cluster sizes. In addition, the MD simulations for MS show evidence of large, system-spanning clusters at lower ϕ . The trend towards aggregation is even more pronounced for LS, where the GCMC simulations suggest a tendency for particles to coalesce into few large clusters (at the expense of clusters of smaller size). In fact, for LS there is no longer a sharp cutoff in the cluster-size distribution. Hence, small clusters, once nucleated, tend to coalesce rapidly. This is clear from the corresponding MD simulations that show clear evidence for aggregation, even at low-volume fractions ( ϕ =0.052). One question is obviously whether the cluster phase is thermodynamically stable (and, if so, whether it remains so upon changing the potential). In particular, one might envisage a situation where the cluster phase is metastable with respect to crystallization. To estimate the relative stability of the crystalline and the cluster phases, we have computed the chemical potential of the constituent hydrate particles both in the cluster phase and in the crystalline phase. In these calculations, we kept the temperatures and pressures of the disordered and ordered phases the same. Hence, the relative stability of the two phases is completely determined by the chemical potential. For the crystalline phase, we used thermodynamic integration (Einstein crystal method) to compute the free energy per particle of the crystal as a function of temperature, at constant pressure (the density was chosen such that P ≈0). From the free energy per particle, we directly obtain the chemical potential of the particles in the crystal. 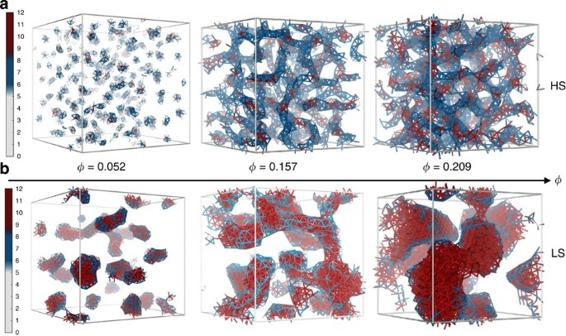Figure 2: Simulation snapshots. Snapshots from MD simulations for HS (a) and LS (b) at different volume fractionsϕandT=0.15. We show only bonds between particles and the colour code indicates the coordination number, varying between 0 (light grey) to 12 (dark red). Table 2 summarizes these results. For the cluster-fluid phase, we determined the chemical potential by using the Widom particle insertion method (see Methods) at volume fractions between ϕ =0.026 and ϕ =0.0104 and pressure ≃ 0. The results are plotted in Fig. 3b,c for HS and LS, respectively, where they are compared with the chemical potential of the crystalline states (black symbols *) obtained from the free energy calculated using the Einstein crystal method and thermodynamic integration (see Methods). For HS the clusters are clearly more stable than the crystalline states. Going to LS instead, the crystalline states have comparable or lower free energies, supporting the idea that in this case the clusters, even though they persist throughout the simulation runs, are only metastable. Figure 2: Simulation snapshots. Snapshots from MD simulations for HS ( a ) and LS ( b ) at different volume fractions ϕ and T =0.15. We show only bonds between particles and the colour code indicates the coordination number, varying between 0 (light grey) to 12 (dark red). 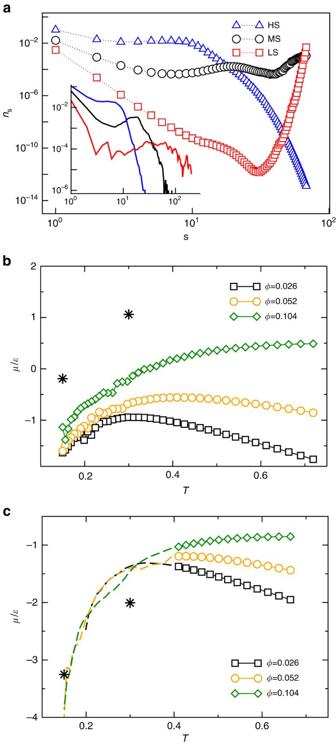Figure 3: Clusters and crystalline states. (a) Cluster size distributionnsfrom GCMC simulations up tos=70 atT=0.25: HS (triangles), MS (circles) and LS (squares). The inset displaysnsat the sameTobtained from the MD simulations atϕ=0.052 forN=6912 particles. The lines are a guide to the eye. (b,c) The values of the chemical potential of the cristalline states (asterisks) fromTable 2are compared with the one in the cluster phase at different volume fractions, computed by Widom insertion for HS (b) and LS (c), as a function of temperature. The dashed lines increfer to the values measured in the region of coexistence of gas and crystalline clusters. Full size image Figure 3: Clusters and crystalline states. ( a ) Cluster size distribution n s from GCMC simulations up to s =70 at T =0.25: HS (triangles), MS (circles) and LS (squares). The inset displays n s at the same T obtained from the MD simulations at ϕ =0.052 for N =6912 particles. The lines are a guide to the eye. ( b , c ) The values of the chemical potential of the cristalline states (asterisks) from Table 2 are compared with the one in the cluster phase at different volume fractions, computed by Widom insertion for HS ( b ) and LS ( c ), as a function of temperature. The dashed lines in c refer to the values measured in the region of coexistence of gas and crystalline clusters. Full size image Table 2 Thermodynamic integration. Full size table In all cases, the shapes of the clusters change with their size: small clusters tend to be roughly spherical, whereas larger clusters are more elongated. A quantitative measure of the elongation is given by the normalized asphericity (see Methods), which equals zero for a spherically symmetric object, +1 for a needle and −0.5 for a disk. The dependence of the asphericity on the cluster size is plotted in Fig. 4a . The data show that upon going from the HS to the LS potential the asphericity decreases: small- and intermediate-size clusters have a fibrillar shape in HS and MS, whereas they are much more spherical in LS, where the asphericity emerges only for much larger clusters (see Supplementary Fig. 1 ). Analysis of the particle arrangements inside the aggregates reveals that the (metastable) clusters for the LS case are quite crystalline (see Supplementary Fig. 2 ). The rotational invariants and computed from the local bond orientational order (BOO; see Methods) [39] allow us to distinguish face-centred cubic (fcc) or hexagonal close-packed (hcp) crystals from the orientational order typical of Bernal spirals (BS), which is compatible with the fibrillar growth of the clusters in HS and MS. 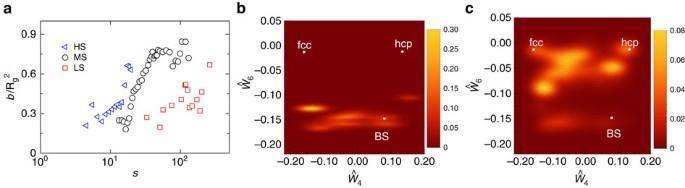Figure 4: Cluster morphology and local order. (a) Asphericity parameter, computed from the gyration tensor of the clusters, as a function of the cluster size atϕ=0.052 andT=0.15 for HS, MS and LS. (b) Heat maps of (,) values atϕ=0.079 andT=0.15 for HS and LS (c). Figure 4b shows indeed that the nature of the local packing in the LS clusters is quite different from that in the HS clusters: for the LS potential, the local packing in clusters appears to fall in the fcc–hcp range, whereas the HS clusters have a structure that is more similar to that of a BS, typical of a fibril-like growth [40] (see Supplementary Figs 3 and 4 ). Figure 4: Cluster morphology and local order. ( a ) Asphericity parameter, computed from the gyration tensor of the clusters, as a function of the cluster size at ϕ =0.052 and T =0.15 for HS, MS and LS. ( b ) Heat maps of ( , ) values at ϕ =0.079 and T =0.15 for HS and LS ( c ). Full size image Arrested states and hydration kinetics Upon increasing the volume fraction of hydrate particles, the clusters grow and interconnect into a gel. The morphology and local packing of this gel also depends on shape of the interaction potential. For HS potential, the fibrillar crystals that are stable at low densities easily grow into a system-spanning network at relatively low-volume fractions, allowing for early development of mechanical properties. Upon decreasing the intermediate-range repulsion towards LS, the fibrils are progressively substituted by large dense and crystalline clusters coexisting with a gas phase. These large clusters can form system-spanning arrested states only at higher-volume fractions (with respect to HS) while favouring the growth of extended and homogeneous high-density regions in the material. The observed equilibrium and arrested states are summarized in the diagrams of Fig. 5 . The solid blue line in HS marks the onset of the geometric percolation of the fibrillar clusters (see Supplementary Fig. 5 ). Along the dashed lines, energy fluctuations measured in MD simulations (NVT, i.e. at constant number of particles N, volume V, and temperature T), display a very weak maximum for HS, as breaking and reforming fibrillar clusters become persistent, and a rather sharp peak in LS, as clusters form from the gas phase, suggesting for LS some kind of coexistence (gas–solid or gas–liquid; see Supplementary Fig. 6 ). The analysis of equilibrium and arrested states discussed so far indicates that packing, local density and morphology changes can occur in the assembly of C–S–H nanoparticles because of changes in the effective interactions during cement hydration (from HS to LS), characterized by a continuous increase in the lime concentration due to the dissolution of the cement grains. As the lime concentration increases, the electrostatic repulsion between the nanoscale hydrates is progressively screened [16] (that is, going from HS to LS). In our model, we assumed that the C–S–H nanoscale units are monodisperse. This is of course an oversimplification: although these nanoclusters have a characteristic size, they seem to be closer to platelet than spheres and tend to be quite polydisperse [11] , [31] , [41] , [42] . Size and shape polydispersity is likely to decrease the stability and predominance of any crystalline structure. However, we expect that the overall aggregation, gelation and densification scenarios discussed above still apply. Aggregate morphologies very similar to the ones discussed here in our equilibrium simulations were indeed observed in nonequilibrium simulations mimicking the precipitation and densification of C–S–H gels with the same effective interactions [43] , [44] . As a matter of fact, the anisotropic growth characteristic of the HS regime, followed by branching, and the densification/rigidification favoured by an evolution towards MS and LS can be directly associated to hallmark steps in cement hydration, corresponding to different stages of the kinetics. Figure 6a shows the hydration curve measured via calorimetry (reprinted from ref. 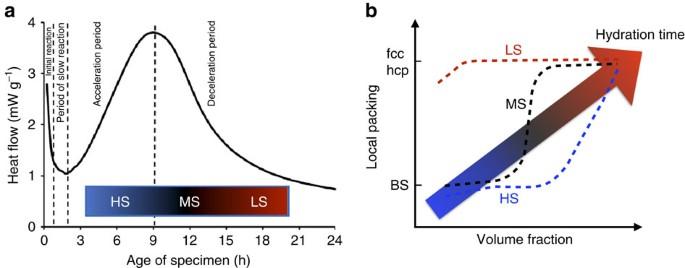Figure 6: Hydration kinetics and nanoscale interactions. (a) The hydration rate as measured via calorimetry during cement hydration reprinted from ref.6(with permission from Elsevier, published subscribed access). It displays the acceleration, deceleration and further densification regime of the kinetics. The colour bar indicates the corresponding evolution of the effective interactions from HS to LS. (b) Schematic drawing of pathways to mechanical strength. To achieve optimal mechanical strength, cement hydrates should first form an open percolating network that can act as a scaffold to form homogeneous dense structures (see text). The figure shows the aggregation pathways (dashed lines) observed in our simulations of HS (blue), MS (black) and LS (red), whereas the arrow indicates a possible pathway during cement hydration. The axis of local packings measures the transition from fibrillar (for example, BS) to compact (fcc/hcp) structures while the system densifies (increasing the volume fractionϕ). As can be seen from the figure, repulsive interactions (HS or MS) are essential for forming the open, fibrillar scaffold. Subsequently, these structures form more compact (fcc or hcp) structures. The transition to a mainly attractive (LS) potential favours hcp. However, the LS potential alone cannot form the low-density fibrillar network and would therefore lead to the formation of heterogeneous high-density structures. 6 ): the colour bar indicates the possible evolution of the effective interactions over time [16] . The early times, corresponding to lower lime concentrations and HS interactions, are characterized by an accelerating regime corresponding to the growth of fibrils that rapidly lead to branching and percolation. The space-filling gel slows down the kinetics and the deceleration regime follows: however, it corresponds to a change towards LS, which favours further densification. Summarizing our findings, the plot in Fig. 6b illustrates the pathways to mechanical strength ( Supplementary Fig. 7 shows a more detailed analysis). To achieve optimal mechanical strength, cement hydrates should first form an open percolating network that can act as a scaffold to form homogeneous dense structures through the densification pathways. The dashed lines depict the sequences of equilibrium structures upon densification at fixed interaction potentials (HS: blue, MS: black, LS: red), whereas the arrow with the changing background colour indicates a possible nonequilibrium pathway with time-varying interactions from HS to MS and LS, consistent with the experiments in ref. 16 . Such a pathway can be manipulated by controlling the chemical composition and its evolution before and during hydration. Building on the results obtained here, one could quantitatively explore the consequences, for the morphology and the mechanical properties, of a different evolution of the effective interactions by suitably designed nonequilibrium simulations. The Supplementary Movie 1 issued from preliminary simulations serves as a proof of concept. These ideas call for a systematic analysis of how changing chemical composition of the dissolving cement and/or chemicophysical conditions (that is, controlling pH, temperature or using various additives) may change the nanoscale effective interactions during hydration as well as their evolution in time. Such an analysis would benefit from experimental, theoretical and simulations combined efforts. 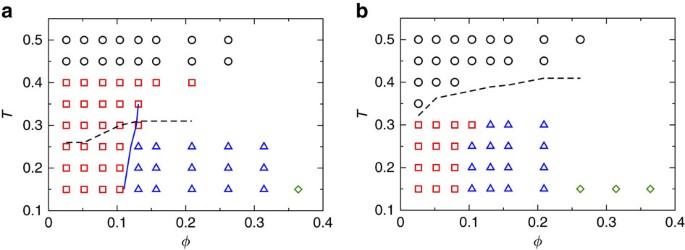With such an analysis at hand, our approach would allow for quantitative predictions of which chemicophysical modifications of C–S–H and cement hydration can enhance strength development, final mechanical performance and durability. Figure 5: Summary of the observed phases. The circles indicate the gas phase, the squares the clusters, the triangles the gel states and the diamonds the crystalline states for HS (a) and LS (b). In HS the solid blue line indicates the geometric percolation of the fibrillar clusters. The dashed lines correspond to the, respectively, weak (for HS) and sharp (for LS) increase in the energy fluctuations measured in MD (NVT) simulations (seeSupplementary Fig. 6). Figure 5: Summary of the observed phases. The circles indicate the gas phase, the squares the clusters, the triangles the gel states and the diamonds the crystalline states for HS ( a ) and LS ( b ). In HS the solid blue line indicates the geometric percolation of the fibrillar clusters. The dashed lines correspond to the, respectively, weak (for HS) and sharp (for LS) increase in the energy fluctuations measured in MD (NVT) simulations (see Supplementary Fig. 6 ). Full size image Figure 6: Hydration kinetics and nanoscale interactions. ( a ) The hydration rate as measured via calorimetry during cement hydration reprinted from ref. 6 (with permission from Elsevier, published subscribed access). It displays the acceleration, deceleration and further densification regime of the kinetics. The colour bar indicates the corresponding evolution of the effective interactions from HS to LS. ( b ) Schematic drawing of pathways to mechanical strength. To achieve optimal mechanical strength, cement hydrates should first form an open percolating network that can act as a scaffold to form homogeneous dense structures (see text). The figure shows the aggregation pathways (dashed lines) observed in our simulations of HS (blue), MS (black) and LS (red), whereas the arrow indicates a possible pathway during cement hydration. The axis of local packings measures the transition from fibrillar (for example, BS) to compact (fcc/hcp) structures while the system densifies (increasing the volume fraction ϕ ). As can be seen from the figure, repulsive interactions (HS or MS) are essential for forming the open, fibrillar scaffold. Subsequently, these structures form more compact (fcc or hcp) structures. The transition to a mainly attractive (LS) potential favours hcp. However, the LS potential alone cannot form the low-density fibrillar network and would therefore lead to the formation of heterogeneous high-density structures. Full size image The simulations presented in this paper provide new insight into how the underlying chemistry of cement formation allows this material to attain its unique mechanical strength, and explain how the natural time evolution of the interactions between hydrate nanoparticles is crucial for attaining the mechanical strength. As the hydrate concentration increases, the repulsion between the nanoparticles gets weaker and densification sets in through thickening of the strands of the gel. This thickening results in increased mechanical strength. Importantly, as gel formation already takes place at low-volume fractions with HS, the densification happens uniformly throughout the system. This is important for the development of mechanical strength: if the densification were to take place through phase separation involving large droplets or crystallites, the resulting material would lack the cohesion that is crucial for its mechanical strength. Moreover, the evolution of the chemical environment that progressively screens electrostatic repulsion as in LS ends up favouring further the continuous densification of the material and hence the development of the mechanical strength needed for construction materials. Understanding the mechanism by which cement is able to attain its unique mechanical strength is important for the rational design of novel, cement-like construction materials. The implication is a novel perspective and opportunity to start designing the hydration process and material properties. By providing new fundamental understanding, our study gives a proof of principles of how controlling and changing the chemical composition and the time evolution of the chemical environment can become the handles for a scientifically guided material design of cements. While indicating a novel investigation path for nanoscale research in cement, our work provides a new opportunity to bridge the microscopic features of the material with the engineering-scale description as attempted in refs 45 , 46 , 47 . The same insights could also be used profitably to achieve high mechanical strength in other (for example, polymeric) materials that can be formed by nanoparticle aggregation. MD and Monte Carlo simulations We have investigated the three cases (LS, MS and HS) by MD simulations in the microcanonical (NVE, i.e., at constant number of particles N, volume V and energy E) and canonical (NVT) ensemble using a Nosé–Hoover thermostat [48] . Initial configurations of 2,048 and 6,912 particles were prepared at different fixed-volume fractions by varying the simulation box size (from L box =13.679 σ to L box =51.706 σ ), at high relative temperature ( T =1), and slowly cooled to carefully equilibrate them at T =0.15. We used a time step δt =0.0025 for the MD, with up to 10 7 steps for thermalization. All the results presented from the MD simulations are averaged over five independent samples. From the particle number density ρ we estimate the fraction ϕ of the total volume occupied by particles as approximately ϕ ≃ ( π /6) ρσ 3 . Most of the simulations were performed by LAMMPS [49] . We have monitored internal energy, kinetic energy and different time-correlation functions, which did not show any significant aging up to ϕ ≃ 0.15. For ϕ >0.15 the thermalization requires increasingly longer times and in the simulations we obtained arrested states that depend on the thermalization protocol and on the system size. In order to sample more efficiently the equilibrium phases, we have performed parallel tempering Monte Carlo (MC) simulations [50] . We simulated M =40 replicas of the same system at different temperatures T 1 ,…, T M . The replicas’ temperatures range from T 1 =0.15 to T M =0.7 in such a way that the two adjacent temperatures differ by a factor of T i +1 / T i =1.04. Replicas are either randomly initialized or initialized from the MD configurations equilibrated at the corresponding temperatures. For each replica we perform the same number of MC steps at a given temperature using MC moves of individual particles as well as cluster moves, that is, translation moves of all the particles that belong to the same cluster. Cluster moves that result in cluster fusion are rejected. We attempt to swap particle configurations between two adjacent replicas i and i +1 with the prescribed Metropolis-based probability [50] , where T i and T i +1 are the temperatures and U i and U i +1 are the total potential energies of the two replicas. In order to achieve sufficient swapping acceptance between replicas, the average energy difference between the adjacent replicas U i − U i +1 need to be comparable to energy fluctuations. Since expected energy U i scales linearly with the number of particles N , whereas the corresponding fluctuations as , the larger the number of particles the smaller the temperature difference between the adjacent replicas needed to be, that is, more replicas are needed to cover the desired temperature range. Therefore, for MC we have used a smaller number of particles ( N ≃ 500). This enables for a successful replica-swapping with acceptance probabilities of ∼ 0.10–0.3, which is considered an optimal choice [51] . We performed simulations with 20–80 × 10 6 MC steps, using the first half for equilibration and the second half for sampling. The percolation thresholds just reported depend on the temperature and also on the cooling protocol used for the systems at different T and ϕ . They have been evaluated for a fixed system size; hence, they are not intended to be exact by any means, since this would require a finite-size scaling analysis. The arrested states discussed here depend of course on the specific kinetic path selected by the MD simulations, that is, they are specific of the NVE or NVT MD simulations performed and of the cooling protocol chosen. We have verified that, for sufficiently slow cooling, the gel morphology and properties discussed here are not significantly affected by the cooling rate. They could change if MD simulations were performed at constant pressure (rather than at constant volume), although we have monitored the pressure in our simulations and we could not detect any steep or abrupt change in pressure upon gel formation. On this basis, we do not expect too large differences. With respect to experimental conditions, one could expect gelation to result into the development of tensile internal stresses because of the net attractive interactions that drive the gelation and to the formation of a poorly connected structure. Hence, the periodic boundary conditions and the imposed fixed volume used for the MD simulations could share some similarities with the experimental conditions under which gels are forming. Free energy calculations We have used a reversible path between the solid obtained in the simulations and an ideal Einstein crystal with the same structure [52] , [53] . The ideal Einstein crystal consists of particles attached to their lattice positions via harmonic springs of constant Λ E , and its free energy A 0 ( T , ρ ) can be analytically evaluated. The free energy difference, Δ A 1 ( T , ρ ), between the ideal Einstein crystal and the interacting Einstein crystal (in which particles interact through the interparticle potential used in the simulations) can be expressed as where U lattice is the potential energy of the perfect lattice and U s the potential energy of the solid obtained in the simulations with the given interparticle interactions. The free energy difference between the interacting Einstein crystal and this solid Δ A 2 ( T , ρ ) can be computed as where the integrand is the mean square displacement of particles from their lattice positions. To calculate Δ A 1 ( T , ρ ) and Δ A 2 ( T , ρ ), we performed canonical (NPT, i.e. at constant number of particles N, pressure P and temperature T) MD simulations of 2,048 particles at zero pressure and different temperatures using LAMMPS [49] , [54] . From Δ A 1 ( T , ρ ) and Δ A 2 ( T , ρ ), we get the free energy of the solid obtained in the simulations as Additional thermodynamic information has been obtained by measuring the chemical potential using the Widom insertion method [55] . The total chemical potential μ of interacting particles is composed of two parts, with the first term corresponding to an ideal gas contribution of density ρ , and μ exc being the excess part due to the presence of particle–particle interactions. For the purpose of test particle insertions, we used particle configurations obtained by the MC simulations. From the resulting potential energies, U i of the inserted particle at random positions (2 × 10 6 per sampled snapshot), the excess chemical potential can be evaluated from where 〈…〉 denotes the average over all particle positions over the whole sampled trajectories. Owing to the lower repulsion, LS crystals have much lower free energy than the HS ones (The free energies of the fcc and hcp crystals are the same within the error bar of our calculation; therefore, we cannot distinguish which crystal is more stable.). Grand canonical simulations As already mentioned, in cases of low ϕ we obtain persistent clusters whose nature, stable or metastable, is difficult to discriminate. To elucidate this point, we have also evaluated the cluster-size distribution by free energy calculation using GCMC simulations. We followed the same procedure introduced to investigate micelle formation in refs 56 , 57 . In an approximation of a dilute gas of clusters, such that interactions between the clusters are negligible, we can decompose the total partition function of the system into contributions of individual clusters where N s is the number of clusters with size s , V is the volume of the system and Q s is the single cluster (of size s ) partition function. We have ignored the (irrelevant) factor because of the thermal de Broglie wavelength. Upon minimizing the total free energy − k B T log Q with respect to cluster size N s , with the constraint of total number of particles , one obtains the number of clusters of size s in equilibrium, The related cluster-size distribution is therefore n s = N s / N cl , where corresponds to the total number of clusters in the system. This yields with ρ = N / V being the particle number density. The parameter plays the role of the chemical potential in a diluted system with β =1/ k B T , and the parameters n 1 = N 1 / N cl and are fixed by the two constraints The ratio of partition functions Q s / Q 1 is computed in the GCMC simulations. As in the MC simulations, we implemented a parallel tempering scheme, but limited the simulations to one single cluster by rejecting all the moves that would break the cluster. That is, besides particle translation moves as in usual MC, we also performed insertions and deletions of particles according to the standard GCMC scheme with the restriction to preserve a single cluster in the system, that is, only insertions within the attractive wells of particle interactions were attempted. Here the volume in the standard GCMC acceptance rule for the particle insertion corresponds to the total volume of all attractive wells. In order to preserve detailed balance, in case of overlap of k attractive wells of neighbouring particles at the location of an insertion attempt, the standard insertion acceptance probability needs to be corrected (multiplied) by a factor 1/ k . During the simulation, we were sampling the probability distribution of the single cluster size P ( s ), which is related to the ratio of the partition functions as where μ GC is an arbitrary value used in the simulations for the chemical potential, which does not affect the ratio Q s / Q 1 but influences the sampling efficiency. The chemical potential μ GC used in GCMC should not be confused with in equation (10). In order to further increase sampling efficiency, we have implemented the standard Umbrella Sampling scheme where we sample at once a cluster of only two possible sizes, s and s +1. The results for all cluster sizes are obtained by stitching together the simulation results of different cluster sizes [57] . Observables The radial distribution function g ( r ) is defined as where N is the number of particles and ρ their density. We define a cluster as a group of those particles that are mutually separated by r ≤ r c , where r c is distance of the minimum followed by the first peak in g ( r ). As the aggregation proceeds, we sample the cluster-size distribution as the number of clusters n s composed of s particles. To characterize the morphology of such clusters, we determine the gyration tensor where N s is the total number of cluster of s particles, is the a th coordinate of the position vector r i of the i th particle belonging to the cluster j and is the a th coordinate of the position of the centre of mass of cluster j . The gyration radius is defined as the sum of the eigenvalues of the gyration tensor: where the eigenvalues of S ab ( s ) are sorted in descending order, that is, λ 1 ≥ λ 2 ≥ λ 3 . In addition, the asphericity parameter measures the deviation from the spherical symmetry ( b =0). Finally, the BOO parameters enable us to characterize the local order [39] . The BOO are defined as where is the number of the bonded neighbours of particle i (using the cutoff distance r c ). The unit vector specifies the orientation of the bond between particles i and j . The are the corresponding spherical harmonics. The second-order rotational invariants and the normalized third-order invariants with (where the coefficients in the sum are the Wigner 3-j coefficients) can be used to identify specific orientational order. In fact, the first non-zero (apart from l = m =0) as found in systems with cubic symmetry for l =4 and in systems with icosahedral symmetry for l =6. The BOO parameters ( ) are generally sufficient to characterize orientational order typical of crystalline solids, colloidal gels and glasses. We use and , as they are sufficient to characterize the local order of interest and distinguish between fcc and hcp crystals. We compute the BOO locally for each particle within the cutoff distance r c . Data availability The authors declare that all data supporting the findings of this study are available within the article and its Supplementary Information Files . How to cite this article: Ioannidou, K. et al . The crucial effect of early-stage gelation on the mechanical properties of cement hydrates. Nat. Commun. 7:12106 doi: 10.1038/ncomms12106 (2016).